The genetic basis of cytoplasmic male sterility and fertility restoration in wheat Hybrid wheat varieties give higher yields than conventional lines but are difficult to produce due to a lack of effective control of male fertility in breeding lines. One promising system involves the Rf1 and Rf3 genes that restore fertility of wheat plants carrying Triticum timopheevii -type cytoplasmic male sterility (T-CMS). Here, by genetic mapping and comparative sequence analyses, we identify Rf1 and Rf3 candidates that can restore normal pollen production in transgenic wheat plants carrying T-CMS. We show that Rf1 and Rf3 bind to the mitochondrial orf279 transcript and induce cleavage, preventing expression of the CMS trait. The identification of restorer genes in wheat is an important step towards the development of hybrid wheat varieties based on a CMS- Rf system. The characterisation of their mode of action brings insights into the molecular basis of CMS and fertility restoration in plants. Genetic improvements in crop performance are crucial for increasing crop productivity, but current rates of improvement will not be sufficient to meet future food demands in an era of global climate change [1] , [2] , [3] . As arable land is limited, increased crop productivity must come from yield increases achieved by innovation in plant breeding [4] , [5] , [6] . By providing 20% of global dietary energy, wheat is one of the most important grain crops cultivated worldwide [7] , [8] , and together with maize and rice contributes 70% of global crop production [9] . However, while rice and maize yields have benefitted strongly from the use of hybrids to exploit heterosis, hybrid wheat varieties are not produced on a commercial scale, even though the estimated yield improvements could reach 20% in a context of climate change and increased disease pressure [10] , [11] , [12] . The lack of hybrid development has restricted the rate of wheat yield gain over the last two decades compared to yield gains in maize or rice [8] , [13] . Hybrid production in autogamous plants requires a method to block self-pollination [14] . A system that has been used for production of hybrids in many crop plants including maize, rice and sorghum is based on cytoplasmic male sterility (CMS), a mitochondrially-encoded trait [15] , [16] , [17] , coupled with one or more nuclear Restorer-of-fertility ( Rf ) genes able to suppress CMS in F 1 plants [14] . This breeding system exploits the genes controlling gynodioecy in natural populations of many flowering plants. Effective CMS sources have been discovered in wheat, such as T-CMS derived from a cross between Triticum timopheevii Zhuk. as female parent and bread wheat as the male parent [18] . However, a lack of effective Rf genes has been a major factor limiting the application of CMS to hybrid seed production in wheat [13] . Based on studies in other plant species, it is known that Rf proteins are encoded in the nucleus and post-translationally imported to mitochondria, where they generally prevent the accumulation of gene products from CMS-specific open reading frames (ORFs) [17] , [19] , [20] . The majority of Rf genes in higher plants encode RNA-binding pentatricopeptide repeat (PPR) proteins [14] , [21] , [22] . The wheat genome contains a surprisingly large number (over 200) of Restorer-of-fertility-like ( RFL ) genes, the majority of which are organised in clusters on chromosomes 1, 2 and 6 [23] . Several Rf genes controlling fertility in the T-CMS system have been reported in Triticum aestivum L. that map to these RFL clusters, including Rf1 (chr1A) [24] , [25] , [26] , [27] and Rf3 (chr1B) [28] , [29] , [30] , [31] , [32] , [33] . Here, we report the identification of Rf1 and Rf3 as PPR proteins and demonstrate their ability to suppress T-CMS in wheat by transgenesis. Both proteins bind to and induce cleavage of transcripts of a previously unrecognised mitochondrial gene ( orf279 ) with no impact on the processing of orf256 , the gene previously thought to cause male sterility in wheat. Mapping of the genomic regions harbouring Rf1 and Rf3 restorer genes We analysed three F 2 mapping populations (R197xKalahari, R204xAlixan and R0932ExAltigo) segregating for Rf1 and three F 2 mapping populations (TJB155xAnapurna, 2852xAltamira, and AH46xR0946E) segregating for Rf3 . Fine mapping by analysis of the progenies of recombinant plants defined the Rf1 interval to be a region between 7.5 and 8.8 cM on chromosome 1A (Fig. 1a ), and the Rf3 interval to be between 22.2 and 22.7 cM on chromosome 1B (Fig. 1b ). The International Wheat Genome Sequencing Consortium (IWGSC) RefSeq v1.0 assembly [23] was used to anchor these intervals to genome sequence scaffolds (Fig. 1 ). Fig. 1: Genetic map of the Rf1 and Rf3 loci in wheat Chinese Spring. a The genetic markers delimiting the Rf1 interval on chromosome 1A (chr1A) were genotyped and mapped in three populations segregating for male-fertility restoration conferred by the Rf1 gene. The 0.8 Mbp region delimited by marker cfn0522096 and cfn0527067 is indicated and the RFL genes present in the interval are shown. b The genetic markers delimiting the Rf3 interval on chromosome 1B (chr1B) were genotyped and mapped in three populations segregating for Rf3 and a doubled-haploid line carrying the Rf3 gene. The 2.8 Mbp region delimited by marker cfn1249269 and BS00090770 is indicated and the RFL genes present in the interval are shown. Scaffold sequences were obtained from the URGI IWGSC sequence repository ( https://wheat-urgi.versailles.inra.fr/ ). Gene sequences that are truncated or disrupted by a frameshift are indicated by lighter colouring. The proposed order of the genes in the Rf3 interval in the Rf3 and Fielder line is only approximate. cM centimorgan, Mbp megabase pair. 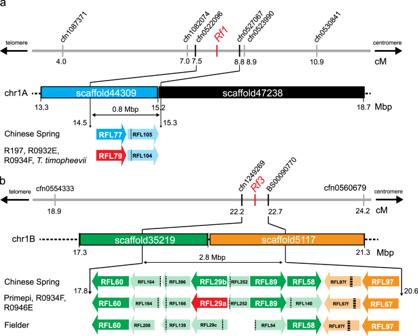Fig. 1: Genetic map of theRf1andRf3loci in wheat Chinese Spring. aThe genetic markers delimiting theRf1interval on chromosome 1A (chr1A) were genotyped and mapped in three populations segregating for male-fertility restoration conferred by theRf1gene. The 0.8 Mbp region delimited by marker cfn0522096 and cfn0527067 is indicated and the RFL genes present in the interval are shown.bThe genetic markers delimiting theRf3interval on chromosome 1B (chr1B) were genotyped and mapped in three populations segregating forRf3and a doubled-haploid line carrying theRf3gene. The 2.8 Mbp region delimited by marker cfn1249269 and BS00090770 is indicated and the RFL genes present in the interval are shown. Scaffold sequences were obtained from the URGI IWGSC sequence repository (https://wheat-urgi.versailles.inra.fr/). Gene sequences that are truncated or disrupted by a frameshift are indicated by lighter colouring. The proposed order of the genes in theRf3interval in theRf3and Fielder line is only approximate. cM centimorgan, Mbp megabase pair. The marker sequences are listed in Supplementary Table1. The marker sequences are listed in Supplementary Table 1 . Full size image RFL genes present in the Rf1 and Rf3 intervals in the wheat reference genome In the IWGSC RefSeq v1.0 reference genome [23] , 13 genes are annotated in the Rf1 interval of which two are RFL-type PPR genes. In the slightly larger Rf3 interval, 28 genes are present, nine of which are RFL-type PPR genes (Fig. 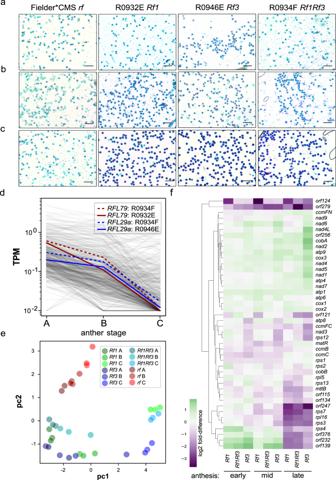Fig. 2: Expression profiles of nuclear and mitochondrial genes in fertile and sterile wheat genotypes during anther development. Alexander’s staining of viable and non-viable pollen grains from anthers collected at three developmental stages: early heading (a), early/mid anthesis (b) and late anthesis (c). Scale bar = 200 μm. This experiment was performed twice. A representative from 20 micrographs for each genotype is shown.dExpression profile ofRFLgenes in three wheat genotypes: R0932E carryingRf1, R0946E carryingRf3and R0934F carryingRf1andRf3. The expression profiles ofRFL79andRFL29a—the two candidates forRf1andRf3—are highlighted in blue and red, respectively. TPM: Transcript per million values calculated from RNA-Seq data. Anther stages A, B and C correspond to the three developmental stages of anther development as described in (a–c).ePrincipal components analysis (PCA) of the read counts for 44 mitochondrial transcripts. The first principal component (pc1, 65% of variance) distinguishes between the three stages in the fertile genotypes and the second principal component (pc2, 14% of variance) distinguishes the fertile and sterile genotypes.fHierarchical clustering of 44 mitochondrial transcripts based on read counts in fertile lines relative to the sterile line at the equivalent developmental stage calculated from RNA-Seq data.Rf1= R0932E,Rf3= R0946E,Rf1Rf3= R0934F. Early, mid and late anthesis correspond to the three developmental stages of anther development as described in (a–c). This experiment was performed once. Three biological replicates each comprising 15 anthers from 3 to 4 individual spikelets were used for RNA extraction and the expression analysis. Source data underlying Fig. 2a–c are provided as a Source data file. Data and code used to generate the plots in Fig. 2d–f are obtainable from Dryad88. 1 , Supplementary Table 2 ). Of the two RFL genes identified in the Rf1 interval on chromosome 1A, only one encodes a full-length PPR protein; the other is truncated at the C-terminus (Fig. 1a , Supplementary Table 2 ). The Rf3 interval on chromosome 1B includes five full-length RFL genes, three truncated RFL genes and one frame-shifted RFL open reading frame (Fig. 1b , Supplementary Table 2 ). The full-length RFL sequences present in the intervals are composed of 741–790 codons and 17–19 PPR motifs (Supplementary Table 2 ). TargetP v1.01 [34] identified a mitochondrial targeting peptide (mTP) (Supplementary Table 2 ) at the N-terminus of the majority of the proteins. Enrichment and sequencing of RFL genes in T. timopheevii and eight wheat accessions The T. aestivum Chinese Spring accession from which the reference genome was obtained is classified as a partially restoring genotype containing a weak Rf3 allele [35] . To identify Rf1 and Rf3 candidates from restoring genotypes without the need for full genome sequencing and assembly, a customised RFL capture approach was developed. 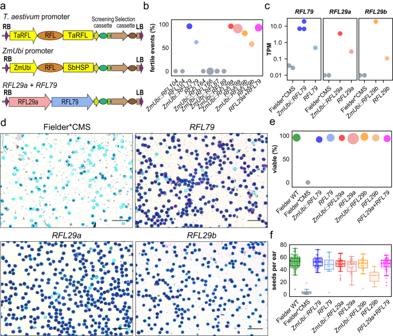Fig. 3: Transformation ofRf1andRf3candidate genes into the Fielder*CMS line. aDesign of the constructs used in plant transformation experiments.TaRFL, sequence from the wheatRfcandidate gene;ZmUbi,Zea maysubiquitin promoter;SbHSP, 3′-UTR fromSorghum bicolorheat shock protein gene. The screening cassette consists of theT. aestivumHMWG gene promoter,ZsGreencoding sequence andtNosterminator sequence. The selection cassette consists of a rice actin gene promoter, thebialaphos resistance(Bar) gene andtNosterminator sequence. RB right border, LB left border.bEvaluation of fertility restoration byRf1andRf3candidates based on the percentage of T0events giving fertile plants. The area of the plot markers is proportional to the total number of transformation events obtained, ranging from 13 to 69.cExpression level of the restoring transgene in transcript per million (TPM) values calculated from RNA-Seq data. The values shown are TPM + 0.01 to allow the Fielder*CMS results to be plotted on a log scale; all three of these genes are absent from Fielder and undetected in the cases of theRFL29aandRFL29b; a few reads mapped toRFL79indicating a low level of cross-mapping from related RFL genes.dAlexander’s stain of pollen grains collected from anthers at late anthesis (anther stage C) of Fielder*CMS and restored transformants (T1generation). This experiment was performed once. The selected micrographs are representatives of 10–15 individual images. Scale bar = 200 μm.ePollen viability counts from analysis of 10–15 images like those in (d). The area of the plot markers is proportional to the number of pollen grains counted, ranging from 920 to 5215.fPlant fertility based on seed set per ear on T1plants from five different transgenic events per construct. Number of ears analysed per line: Fielder WTn= 1043, Fielder*CMSn= 125,ZmUbi::RFL79n= 313,RFL79n= 92, ZmUbi::RFL29an= 209, RFL29an= 197, ZmUbi::RFL29bn= 107, RFL29bn= 43, RFL29a+RFL79n= 359. Centre line, median; box limits, upper and lower quartiles; whiskers, 1.5× interquartile range. Source data underlying (b) and (d–f) are provided as a Source data file. Data and code used to generate the plots in panel Fig. 3c are obtainable from Dryad88. DNA baits were designed based on 1199 RFL (PPR) sequences extracted from 33 genomic and two transcriptome data sets from 27 cereal species and their wild relatives (Supplementary Table 3 ). 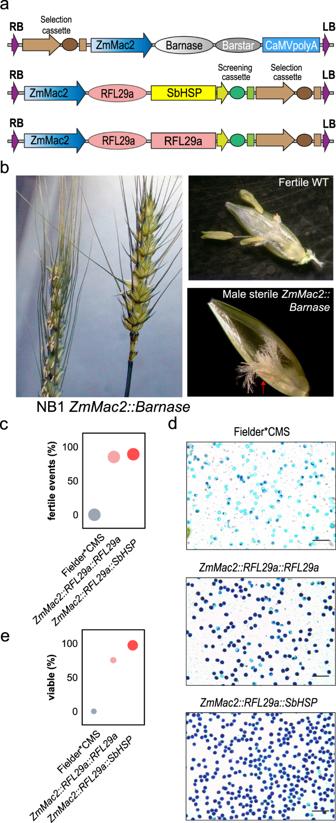Fig. 4: Restoration of fertility byRFL29adriven by a tapetum-specific promoter. aConstructs used in the experiment.bImages showing complete male sterility induced by expression of theZmMac2::Barnaseconstruct in wheat. Red arrow shows aborted anther with only filament.cPlant fertility is restored by expression ofZmMac2::RFL29a. Plot marker area is proportional to the total number of transformation events obtained, ranging from 19 to 20.dPollen fromZmMac2::RFL29aplants stained for viability, showing substantial restoration of normal pollen development. This experiment was performed once. A representative from 20 micrographs is shown. Scale bar = 200 μm.ePollen viability counts. Plot marker areas are proportional to the number of grains counted, ranging from 920 to 3142. Source data underlying Fig. 4b–e are provided as a Source data file. These baits were used to enrich genomic DNA fragments containing RFL sequences from eight wheat accessions and T. timopheevii (Supplementary Table 4 ). The selected DNA fragments were sequenced on an Illumina MiSeq platform. On average, 220 RFL contigs were obtained from each hexaploid T. aestivum accession and 138 from the tetraploid T. timopheevii (Supplementary Table 4 ). For each of the 216 RFL sequences in the Chinese Spring reference genome, a corresponding sequence was obtained by the RFL capture approach with the only differences being due to occasional incomplete assembly of the full reading frame outside of the PPR motifs (Supplementary Table 4 ), confirming the accuracy of the assembly approach used for the captured fragments. Within these contigs, RFL-type ORFs were identified across all nine genotypes. The number of ORFs per accession ranged from 143 in T. timopheevii to 262 in accession R0946E (Supplementary Table 4 ). To identify putatively orthologous RFL sequences, they were grouped using CD-HIT v4.6.4 [36] using a threshold of 96% sequence identity (Supplementary Data 1 ), which we found to be the best compromise between distinguishing paralogous sequences within each accession while grouping putatively orthologous sequences across accessions. Selection of candidate Rf1 and Rf3 orthologous groups We selected candidate Rf1 and Rf3 groups from the 397 orthologous RFL groups based on whether the restoring genotypes contained a putatively full-length, functional member of that group, while the non-restoring genotypes did not. 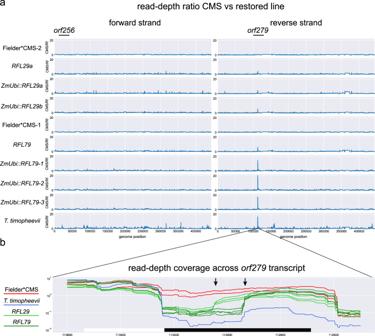Fig. 5: Identification oforf279as a gene associated with T-CMS in wheat. aRatio of strand-specific RNA-Seq coverage from Fielder*CMS lines (sterile) and restored (fertile) samples plotted across theT. timopheeviimitochondrial genome (NCBI accession number NC_022714.1) for forward and reverse strand is shown. The genomic regions carryingorf256(forward strand) andorf279(reverse strand) are indicated at the top of the plots. The number of replicates forZmUbi::RFL29a,ZmUbi::RFL29b, RFL29a,RFL79andT. timopheeviiwasn= 1, Fielder*CMSn= 2 and forZmUbi::RFL79n= 3.bNormalised RNA-Seq coverage in theorf279region.orf279is indicated by the boxes below the chart, distinguishing the part oforf279that is identical toatp8(white box) and theorf279-unique region (black box). The number of RNA-Seq reads mapped to the central region oforf279in restorer line is much lower than in Fielder*CMS. The sharp transition from low to high coverage (arrows) indicates the probable site of RNA cleavage induced by a restorer gene. Data and code used to generate the plots in the panels are obtainable from Dryad88. The list of candidates was refined by excluding those that mapped outside the intervals established by the genetic mapping (Supplementary Table 5 ). In addition, as the Rf1 gene most likely originates from T. timopheevii [24] , [25] , the Rf1 candidate groups should contain a representative from T. timopheevii . On the contrary, Rf3 originates from T. aestivum [33] , therefore the candidate Rf3 groups should not contain an identical representative from T. timopheevii . First, we identified the orthologous RFL groups comprising at least one sequence captured from an accession characterized as carrying the Rf1 gene (accessions R197, R0932E, R0934F and T. timopheevii ) (Supplementary Table 5 ). In silico mapping of the candidate sequences to estimate their genomic location on chromosome 1A was achieved by aligning the DNA contigs to the reference genome. To confirm the location of the candidate RFLs within the Rf1 interval, several gene-specific markers were developed for each gene and genetic mapping was performed (Supplementary Table 5 ). The mapping allowed orthologous RFL groups that mapped outside of the Rf1 interval on chromosome 1A (Supplementary Table 5 ) to be discarded. In this way, four orthologous RFL groups (79, 104, 185 and 268) were identified as potential candidates for the Rf1 gene in wheat (Supplementary Table 5 ). The protein sequences from groups RFL185 and RFL268 are only partial (<500 amino acids long) and correspond to two parts of the same gene that was split by a frameshift (Supplementary Data 1 ). Therefore, both proteins were considered as unlikely to be functional and excluded as candidates for Rf1 . As both RFL79 and RFL104 are composed of 750+ amino acids and ~17 PPR motifs (Supplementary Table 5 ) these two sequences were considered as being the best candidate Rf1 groups. To select candidates for Rf3 , orthologous RFL groups were screened for full-length protein sequences present in the Rf3 -containing Primepi, R0946E and R0934F genotypes but absent from (or partial in) the rf3 genotypes. This analysis allowed the identification of nine candidate groups of which seven were identified to be located within the Rf3 interval by genetic mapping (Supplementary Table 5 ). RFL29 and RFL89 orthogroups encode full-length RFL proteins (Supplementary Table 5 ). Three versions of RFL29 exist within the RFL29 group (Fig. 1b , Supplementary Fig. 1 ). The RFL29a allele is present in Primepi, R0946E and R0934F, the RFL29b allele is found in the weak restorer line Chinese Spring, and the RFL29c version found in Fielder carries an indel that disrupts the coding sequence (Fig. 1b , Supplementary Fig. 1 ). RFL29a and RFL29b are highly similar, with only eight amino acid polymorphisms and two extra amino acids inserted near the N-terminus of RFL29b (Supplementary Fig. 1 ). There is also an insertion in the putative 5′ untranslated region (UTR) of RFL29b (Supplementary Fig. 1 ). This, in addition to the coding sequence polymorphism observed between Rf3 lines and non-restoring accessions, indicated RFL29a as a candidate for Rf3 . The sequences from Rf3 genotypes Primepi, R0946E and R0934F appear to be full-length and putatively functional (Supplementary Table 5 ). In groups RFL67 and RFL89 , the only full-length sequences identified were from Rf3 genotypes. Expression of Rf1 and Rf3 candidates in anthers during pollen formation We looked at gene expression during anther development to see if these Rf1 and Rf3 candidates are expressed during the critical phases when differences between male-sterile and male-fertile genotypes become apparent. Three stages of anther development were chosen as visualized by pollen staining in Fig. 2a–c , and corresponding to early, mid and late anthesis respectively. Based on the use of Alexander’s stain to distinguish viable and non-viable pollen, clear differences between sterile and fertile plants are visible at mid and fully developed by late anthesis (Fig. 2b, c ). Total RNA was extracted from developing anthers at these three stages, depleted of rRNA and sequenced using random hexamer primers to allow unbiased capture of mitochondrial transcripts in addition to cytosolic and nuclear transcripts. Principal components analysis (PCA) of the read counts for each transcript showed strong differentiation between the three stages in the fertile plants (first principal component, Supplementary Fig. 2 ) and strong differentiation between the fertile and sterile genotypes (second principal component, Supplementary Fig. 2 ). The RNA-Seq reads were mapped against the captured RFL contigs for each line to determine expression levels for each RFL gene. Most RFL genes are expressed at low levels (0.1–1 transcript per million) at early anthesis (anther stage A), with the expression level falling by mid anthesis (anther stage B) and often undetectable by late anthesis (anther stage C) (Fig. 2d ). The Rf1 and Rf3 candidates follow this pattern, although with expression levels a little above the median of RFL expression, particularly at mid anthesis (anther stage B). Thus, the Rf1 and Rf3 candidates are expressed in anther tissue in the critical period when pollen formation starts to differ between fertile and sterile lines. Fig. 2: Expression profiles of nuclear and mitochondrial genes in fertile and sterile wheat genotypes during anther development. Alexander’s staining of viable and non-viable pollen grains from anthers collected at three developmental stages: early heading ( a ), early/mid anthesis ( b ) and late anthesis ( c ). Scale bar = 200 μm. This experiment was performed twice. A representative from 20 micrographs for each genotype is shown. d Expression profile of RFL genes in three wheat genotypes: R0932E carrying Rf1 , R0946E carrying Rf3 and R0934F carrying Rf1 and Rf3 . The expression profiles of RFL79 and RFL29a —the two candidates for Rf1 and Rf3 —are highlighted in blue and red, respectively. TPM: Transcript per million values calculated from RNA-Seq data. Anther stages A, B and C correspond to the three developmental stages of anther development as described in ( a – c ). e Principal components analysis (PCA) of the read counts for 44 mitochondrial transcripts. The first principal component (pc1, 65% of variance) distinguishes between the three stages in the fertile genotypes and the second principal component (pc2, 14% of variance) distinguishes the fertile and sterile genotypes. f Hierarchical clustering of 44 mitochondrial transcripts based on read counts in fertile lines relative to the sterile line at the equivalent developmental stage calculated from RNA-Seq data. Rf1 = R0932E, Rf3 = R0946E, Rf1Rf3 = R0934F. Early, mid and late anthesis correspond to the three developmental stages of anther development as described in ( a – c ). This experiment was performed once. Three biological replicates each comprising 15 anthers from 3 to 4 individual spikelets were used for RNA extraction and the expression analysis. Source data underlying Fig. 2a–c are provided as a Source data file. Data and code used to generate the plots in Fig. 2d–f are obtainable from Dryad [88] . Full size image As RFL proteins are expected to have an impact on mitochondrial gene expression, we analysed mitochondrial transcripts in the same RNA-Seq experiment, including not only all the known coding sequences but also ten open reading frames exceeding 100 codons that are only found in the T. timopheevii mitochondrial genome and that could putatively encode CMS-specific polypeptides. Remarkably, PCA analysis on just the 44 mitochondrial transcripts (Fig. 2e ) largely recapitulated the pattern found with 130,404 nuclear and cytosolic transcripts (Supplementary Fig. 2 ), showing the strong correlation between mitochondrial gene expression during anther development and male fertility. Hierarchical clustering of mitochondrial transcripts based on read counts in fertile lines relative to the sterile line (Fig. 2f ) showed a large cluster encoding components of the respiratory chain (complexes I, III, IV and V) that accumulate in the male-fertile lines. In contrast, transcripts for components of the mitochondrial biogenesis machinery (e.g. ribosomal subunits, cytochrome c maturation system) tend to be lower in the fertile lines, particularly by late anthesis. Of the T. timopheevii -specific ORFs, most show lower expression in the fertile lines. The surprising exception is orf256 , whose expression was previously reported to be correlated with T-CMS in wheat [37] , [38] . In contrast, expression of two other T . timopheevii -specific ORFs ( orf124 and orf279 ) is strongly suppressed in the fertile lines. Testing the restoring capabilities of Rf1 and Rf3 candidate genes by transgenesis The coding sequences of RFL79 and RFL104 ( Rf1 candidates) as well as of RFL29a/b , RFL67 , RFL164 , RFL166 and RFL89 ( Rf3 candidates) were cloned into plant transformation vectors under the control of the Zea mays ubiquitin promoter ( ZmUbi ). The RFL104 , RFL79 and RFL29a/b genes were also cloned under the control of their own promoter (Fig. 3a ). The constructs were transformed into a specifically developed Fielder*CMS wheat line—a cultivar harbouring T. timopheevii cytoplasm (T-CMS) but a T. aestivum nuclear genome (‘Fielder’ background) showing high efficiency for Agrobacterium tumefaciens transformation [39] . Transgene insertion in the genome was confirmed by PCR (Supplementary Data 2 ) and the fertility of T 0 transgenic plants was evaluated. No pollen was observed to be produced and no seed set by Fielder*CMS plants or Fielder*CMS plants transformed with RFL104 , RFL164 , RFL166 , RFL89 or RFL67 (Fig. 3b , Supplementary Fig. 3 ). In contrast, fertility was observed in many plants expressing RFL79 or RFL29a/b sequences driven by either their own promoters or the ZmUbi promoter. Fertility restoration was quantitatively evaluated using the frequency of transformation events leading to fertility vs. sterility for each construct (Fig. 3b ). Fertility restoration observed in the T 0 generation for the RFL79 transgene was 96% ( ZmUbi promoter) and 62% (endogenous promoter), respectively. Similarly, the two Rf3 candidates, RFL29a and RFL29b , were observed to confer strong fertility restoration (over 80%) with the ZmUbi promoter. With their endogenous promoters, RFL29a shows better fertility penetrance than RFL29b (Fig. 3b ), in line with a higher level of expression as evaluated by RNA-Seq (Fig. 3c ). A construct combining RFL79 and RFL29a under the control of their own regulatory sequences gave 93% of events showing fertility restoration. Male fertility was investigated more thoroughly in the subsequent generation by staining pollen for viability (Fig. 3d, e ) and counting seeds set per ear and per spikelet (Fig. 3f , Supplementary Fig. 3b ). Fig. 3: Transformation of Rf1 and Rf3 candidate genes into the Fielder*CMS line. a Design of the constructs used in plant transformation experiments. TaRFL , sequence from the wheat Rf candidate gene; ZmUbi , Zea mays ubiquitin promoter; SbHSP , 3′-UTR from Sorghum bicolor heat shock protein gene. The screening cassette consists of the T. aestivum HMWG gene promoter, ZsGreen coding sequence and tNos terminator sequence. The selection cassette consists of a rice actin gene promoter, the bialaphos resistance ( Bar ) gene and tNos terminator sequence. RB right border, LB left border. b Evaluation of fertility restoration by Rf1 and Rf3 candidates based on the percentage of T 0 events giving fertile plants. The area of the plot markers is proportional to the total number of transformation events obtained, ranging from 13 to 69. c Expression level of the restoring transgene in transcript per million (TPM) values calculated from RNA-Seq data. The values shown are TPM + 0.01 to allow the Fielder*CMS results to be plotted on a log scale; all three of these genes are absent from Fielder and undetected in the cases of the RFL29a and RFL29b ; a few reads mapped to RFL79 indicating a low level of cross-mapping from related RFL genes. d Alexander’s stain of pollen grains collected from anthers at late anthesis (anther stage C) of Fielder*CMS and restored transformants (T 1 generation). This experiment was performed once. The selected micrographs are representatives of 10–15 individual images. Scale bar = 200 μm. e Pollen viability counts from analysis of 10–15 images like those in ( d ). The area of the plot markers is proportional to the number of pollen grains counted, ranging from 920 to 5215. f Plant fertility based on seed set per ear on T 1 plants from five different transgenic events per construct. Number of ears analysed per line: Fielder WT n = 1043, Fielder*CMS n = 125, ZmUbi::RFL79 n = 313, RFL79 n = 92 , ZmUbi::RFL29a n = 209 , RFL29a n = 197 , ZmUbi::RFL29b n = 107 , RFL29b n = 43 , RFL29a + RFL79 n = 359. Centre line, median; box limits, upper and lower quartiles; whiskers, 1.5× interquartile range. Source data underlying ( b ) and ( d – f ) are provided as a Source data file. Data and code used to generate the plots in panel Fig. 3c are obtainable from Dryad [88] . Full size image That these genes act through a role in anther development and pollen formation was tested by attempting to restore fertility using RFL29a driven by a tapetum-specific promoter, ZmMac2 (Fig. 4a ). In maize anthers, this promoter is active in the tapetal cell layer during the pollen tetrad stage, with decreasing activity as free microspores are released [40] . Its expression pattern is likely to be similar in wheat, as when used to drive expression of cytotoxic barnase it specifically causes male-sterility, without affecting vegetative or female organ development (Fig. 4b ). Two constructs using ZmMac2 to drive RFL29a expression substantially restored male fertility and pollen formation when used to transform Fielder*CMS (Fig. 4c–e ). Fig. 4: Restoration of fertility by RFL29a driven by a tapetum-specific promoter. a Constructs used in the experiment. b Images showing complete male sterility induced by expression of the ZmMac2::Barnase construct in wheat. Red arrow shows aborted anther with only filament. c Plant fertility is restored by expression of ZmMac2::RFL29a . Plot marker area is proportional to the total number of transformation events obtained, ranging from 19 to 20. d Pollen from ZmMac2::RFL29a plants stained for viability, showing substantial restoration of normal pollen development. This experiment was performed once. A representative from 20 micrographs is shown. Scale bar = 200 μm. e Pollen viability counts. Plot marker areas are proportional to the number of grains counted, ranging from 920 to 3142. Source data underlying Fig. 4b–e are provided as a Source data file. Full size image orf279 is the cause of T-CMS in wheat Previous studies indicated that fertility restoration of T-CMS plants is linked with the expression of Orf256 protein [37] and that the nuclear background influences the processing of the orf256 transcript in wheat accessions [38] . Thus, the expression of orf256 was analysed in RFL79 and RFL29a transformants by RT-PCR (Supplementary Fig. 4 ). The orf256 transcript is detected in both CMS and restored lines (Fig. 2f ) and northern blot analysis revealed that partial cleavage of orf256 RNA already occurs in the sterile Fielder*CMS plants and no additional orf256 cleavage is observed in the fertile Fielder*CMS plants transformed with the ZmUbi::TaRFL79 or ZmUbi::TaRFL29a constructs (Supplementary Fig. 4 ). 5′-Rapid Amplification of cDNA Ends (5′-RACE) analysis confirmed that the cleavage of orf25 6 does not correlate with the restoration of fertility phenotype observed in the transformants (Supplementary Fig. 4 ). Furthermore, northern blot analysis of several wheat accessions carrying T-CMS cytoplasm showed no correlation between the processing of orf256 and the presence of either Rf1 or Rf3 , and cleavage of orf256 is also detected in sterile genotypes (Supplementary Fig. 4d ). As orf256 did not appear to be related to fertility restoration in our material, we carried out a systematic RNA-Seq analysis of RNA samples from Fielder*CMS and restored lines. We observed no significant differences in expression of orf256 (Fig. 5a ) or orf124 (Supplementary Fig. 5 ) but did notice major differences in the expression of a previously unrecognised gene, which we designate orf279 (as the reading frame consists of 279 codons). The 5′ flanking sequence and the first 96 codons of orf279 are identical to atp8 (Fig. 5b ). The remaining 184 codons are contained within a 552 nt sequence present in the T. timopheevii genome but absent from all other sequenced mitochondrial genomes, including the T. aestivum mitochondrial genome (Fig. 5b ). RNA-Seq coverage within part of this unique sequence is lower within the restored plants than in sterile plants. The coverage pattern is consistent with cleavage of orf279 transcripts within the unique region followed by degradation of the 5′ cleavage product and persistence of the 3′ cleavage product (Fig. 5b ). The RNA-Seq data show that the putative 3′ cleavage product is ~110 nt longer in Rf3 plants than in Rf1 plants. This differential processing of orf279 transcripts in RFL79 and RFL29a lines was confirmed by RACE (Supplementary Fig. 6 ). A major 5′-RACE product of ~205 nt was detected in the RFL79 transformants, whereas in RFL29 transformants a major amplicon of ~310 nt was found (Fig. 6a , Supplementary Fig. 6 ). In agreement with the provenance of Rf1 from T. timopheevii and Rf3 from T. aestivum , only the Rf1 -specific 5′-RACE product was detected in T. timopheevii (Supplementary Fig. 6 ). Fig. 5: Identification of orf279 as a gene associated with T-CMS in wheat. a Ratio of strand-specific RNA-Seq coverage from Fielder*CMS lines (sterile) and restored (fertile) samples plotted across the T. timopheevii mitochondrial genome (NCBI accession number NC_022714.1) for forward and reverse strand is shown. The genomic regions carrying orf256 (forward strand) and orf279 (reverse strand) are indicated at the top of the plots. The number of replicates for ZmUbi::RFL29a , ZmUbi::RFL29b, RFL29a , RFL79 and T. timopheevii was n = 1, Fielder*CMS n = 2 and for ZmUbi::RFL79 n = 3. b Normalised RNA-Seq coverage in the orf279 region. orf279 is indicated by the boxes below the chart, distinguishing the part of orf279 that is identical to atp8 (white box) and the orf279 -unique region (black box). The number of RNA-Seq reads mapped to the central region of orf279 in restorer line is much lower than in Fielder*CMS. The sharp transition from low to high coverage (arrows) indicates the probable site of RNA cleavage induced by a restorer gene. Data and code used to generate the plots in the panels are obtainable from Dryad [88] . Full size image Fig. 6: Characterisation of orf279 as genetic basis of T-CMS in wheat. a Comparison of the atp8-1 gene from T. aestivum and orf279 gene from T. timopheevii genome. The gene coding sequences are shown as grey and black boxes. The 5′ and 3′ regions are indicated. The part of orf279 used for production of the Orf279 antibody is indicated by a dashed line. The RNA cleavage sites induced by RFL29a and RFL79, the two candidates for Rf3 and Rf1 restorer in wheat, are shown, and were estimated based on RNA-Seq and 5′ RACE results shown in Supplementary Fig. 6 . b Two transmembrane domains in the Orf279 protein sequence were predicted with TMHMM method [41] on the TMHMM Server v. 2.0 ( http://www.cbs.dtu.dk/services/TMHMM/ ) and are shown in red. TM1 (transmembrane 1) and TM2 (transmembrane 2) encompass amino acid residues 10–29 and 114–136, respectively. TM1 is located within the Atp8 region of Orf279. c Immunological detection of Orf279 in mitochondrial protein extracts. Mitochondrial fractions were enriched from 11-day-old etiolated seedlings grown on vermiculite, treated with n-dodecyl-β-d-maltoside to release membrane-bound proteins and separated on a 15% Stain-Free™ SDS-PAGE gel (Bio-Rad). A Stain-Free image of the gel is shown as a loading control. This experiment was performed three times with similar results. Source data underlying Fig. 6c are provided as a Source data file. Full size image Two transmembrane domains were predicted in the putative orf279 gene product with the TMHMM method [41] (Fig. 6b ). TM1 (transmembrane 1) and TM2 (transmembrane 2) encompass amino acid residues 10–29 (within the Atp8 region) and 114–136 (within the unique region), respectively. A polyclonal antibody directed towards a recombinant protein encompassing the unique part of Orf279 detected a protein of 32 kDa in a mitochondrial protein fraction extracted from Fielder*CMS seedlings but not in equivalent fractions from Fielder or lines transformed with RFL29 or RFL79 (Fig. 6c ). RFL79 and RFL29a bind to the orf279 transcript in vitro The RFL29a and RFL79 proteins were expressed as fusions with a polyhistidine (His) tag and maltose-binding protein (MBP) at the N-terminus (Supplementary Fig. 7 ). Their binding sites within the orf279 transcript (Fig. 7 ) were predicted following the pattern of amino acid combinations at positions 5 and 35 within each PPR motif [42] , [43] . RNA oligonucleotides covering these predicted sites were synthesised and used to test the RNA-binding ability of the two proteins. Both RFL29a and RFL79 bind to their predicted RNA targets within orf279 (Fig. 7 ). More details and caveats on the interpretation of these results are provided in Supplementary Fig. 7 where we show that the majority of the recombinant RFL79 and RFL29a proteins are aggregated. This is likely to negatively influence the RNA-binding ability of the proteins, and may explain why the binding to orf279 RNA probe is weaker than observed for some other PPR proteins (apparent Kd ~ 1 µM compared with 0.1 nM for PPR10 on its favoured target [44] ). Fig. 7: RNA-binding assays with recombinant RFL29a and RFL79 proteins. a Location of the predicted RFL29a and RFL79 binding sites within the orf279 RNA, relative to the observed cleavage sites (red triangles). The predicted binding site for RFL79 encompasses nucleotides 112,975–112,956, and for RFL29a 113,148–113,129 in the T. timopheevii mitochondrial genome (GenBank accession: NC_022714). The key amino acids at positions 5 and 35 of each PPR motif are indicated. The colour scale reflects the strength of the match between the amino acid combination and the RNA base, calculated from in vitro binding data [43] . b RFL29a and RFL79 bind to orf279 as shown by electrophoretic mobility shifts of fluorescein-labelled RNA oligonucleotides corresponding to their predicted targets. B = bound (RNA + protein) U = unbound (free RNA probe). Neither protein binds to an unrelated RNA oligonucleotide (based on orf256 sequence). As both proteins were produced as maltose-binding protein (MBP) fusions, RNA binding with MBP alone was tested and found to be negligible. Serial protein dilutions ranging from 1.8 µM to 28.1 nM for RFL29a and RFL79, and from 0.5 µM to 7.8 nM for MBP were used for the binding assays. The final concentration of the RNA probes was 1 nM. On each gel, the left lane acts as a marker for unbound probe. More details are provided in Supplementary Fig. 7 . 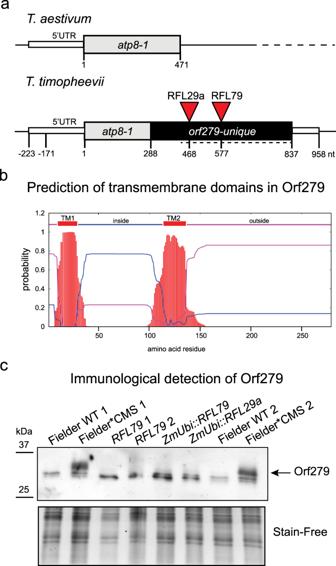Fig. 6: Characterisation oforf279as genetic basis of T-CMS in wheat. aComparison of theatp8-1gene fromT. aestivumandorf279gene fromT. timopheeviigenome. The gene coding sequences are shown as grey and black boxes. The 5′ and 3′ regions are indicated. The part oforf279used for production of the Orf279 antibody is indicated by a dashed line. The RNA cleavage sites induced by RFL29a and RFL79, the two candidates for Rf3 and Rf1 restorer in wheat, are shown, and were estimated based on RNA-Seq and 5′ RACE results shown in Supplementary Fig.6.bTwo transmembrane domains in the Orf279 protein sequence were predicted with TMHMM method41on the TMHMM Server v. 2.0 (http://www.cbs.dtu.dk/services/TMHMM/) and are shown in red. TM1 (transmembrane 1) and TM2 (transmembrane 2) encompass amino acid residues 10–29 and 114–136, respectively. TM1 is located within the Atp8 region of Orf279.cImmunological detection of Orf279 in mitochondrial protein extracts. Mitochondrial fractions were enriched from 11-day-old etiolated seedlings grown on vermiculite, treated with n-dodecyl-β-d-maltoside to release membrane-bound proteins and separated on a 15% Stain-Free™ SDS-PAGE gel (Bio-Rad). A Stain-Free image of the gel is shown as a loading control. This experiment was performed three times with similar results. Source data underlying Fig. 6c are provided as a Source data file. 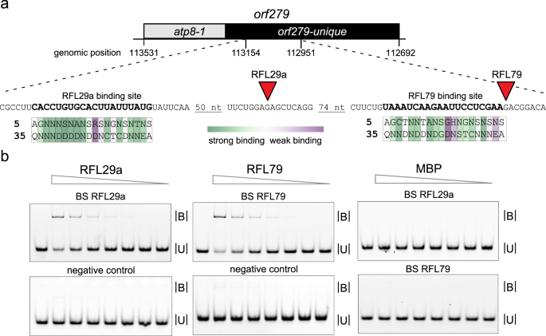Fig. 7: RNA-binding assays with recombinant RFL29a and RFL79 proteins. aLocation of the predicted RFL29a and RFL79 binding sites within theorf279RNA, relative to the observed cleavage sites (red triangles). The predicted binding site for RFL79 encompasses nucleotides 112,975–112,956, and for RFL29a 113,148–113,129 in theT. timopheeviimitochondrial genome (GenBank accession: NC_022714). The key amino acids at positions 5 and 35 of each PPR motif are indicated. The colour scale reflects the strength of the match between the amino acid combination and the RNA base, calculated from in vitro binding data43.bRFL29a and RFL79 bind toorf279as shown by electrophoretic mobility shifts of fluorescein-labelled RNA oligonucleotides corresponding to their predicted targets. B = bound (RNA + protein) U = unbound (free RNA probe). Neither protein binds to an unrelated RNA oligonucleotide (based onorf256sequence). As both proteins were produced as maltose-binding protein (MBP) fusions, RNA binding with MBP alone was tested and found to be negligible. Serial protein dilutions ranging from 1.8 µM to 28.1 nM for RFL29a and RFL79, and from 0.5 µM to 7.8 nM for MBP were used for the binding assays. The final concentration of the RNA probes was 1 nM. On each gel, the left lane acts as a marker for unbound probe. More details are provided in Supplementary Fig.7. Probe sequences are given in Supplementary Table6. This experiment was performed three times with similar results. Source data underlying Fig. 7b are provided as a Source data file. Probe sequences are given in Supplementary Table 6 . This experiment was performed three times with similar results. Source data underlying Fig. 7b are provided as a Source data file. Full size image The potential of hybrid breeding in wheat was recognised by plant breeders at the end of the 19th century [45] . However, this technology has been under-exploited in wheat because of the difficulties in producing hybrids on an industrial scale, despite major efforts from both the commercial and academic sectors [46] , [47] , [48] . Of the different approaches to breeding hybrids that have been explored in wheat [49] , [50] , CMS, so effective in other crops, has been difficult to use because of the genetic complexity and inadequacy of fertility restoration in the hybrids [13] . An understanding of the genetic basis of CMS and fertility restoration in wheat is thus helpful for developing more effective hybrid breeding systems. We followed a positional cloning strategy coupled with a selective sequence capture approach to identify Rf1 and Rf3 , two of the major fertility restorer genes in wheat for T-CMS. Both genes encode members of the RFL clade of the PPR family and reside within large homeologous clusters of related genes. The wheat genome is exceptional in containing more than ~200 RFL genes [23] , compared to 20–30 in a typical plant genome, partially explaining the complexity of fertility restoration genetics in this species. RFL79 ( Rf1 ) and RFL29a ( Rf3 ) are 89% identical in DNA sequence and 83% identical at the protein level (Supplementary Fig. 8 ). Despite this high sequence similarity, and the similar phenotype they are associated with, their molecular action is in fact distinct. RFL proteins are, like other PPR proteins, sequence-specific RNA-binding proteins whose specificity is governed by the amino acid residues at positions 5 and 35 of each PPR motif [42] , [43] . Both RFL79 and RFL29a proteins comprise 20 PPR motifs (Supplementary Fig. 9 ) but their comparison shows that in 13 of these motifs, the 5th/35th amino acid combinations differ between RFL79 and RFL29a. This variation is concordant with previous observations of diversifying selection acting on these residues in RFL proteins [51] , [52] , [53] . RFL29a and RFL79 bind to the orf279 transcript inducing downstream cleavage of the RNA at different sites, leading in both cases to reduced accumulation of the Orf279 protein. Induced cleavage of the targeted transcript at <100 nt 3′ of the RFL-binding site appears to be a general mechanism of action of these proteins [54] . Although it is not unheard of that multiple restorer genes target the same CMS-inducing RNA (e.g. Rf1a and Rf1b in rice [55] , [56] ), this is the first demonstration of two RFL proteins binding the same RNA and inducing its cleavage at different positions. The independent action of Rf1 and Rf3 suggests that stacking the two genes should improve fertility restoration, as indeed we observed (Fig. 3 ). In most cases examined at the molecular level, CMS is correlated with aberrant, usually chimaeric, mitochondrial genes that encode small transmembrane proteins (10–35 kDa) often showing specific spatiotemporal accumulation in anthers or microspores. These proteins are thought to cause a deficiency in ATP production that triggers abnormal programmed cell death in the sporophytic tissues supporting microspore development or in the microspores themselves, ultimately leading to male sterility [14] , [57] . Several CMS-associated ORFs in both monocot and dicot plants contain fragments of conserved mitochondrial genes, often ones encoding subunits of the ATP synthase [14] . In many cases, only circumstantial evidence is available for the link between the presumed CMS-inducing ORF and the male-sterile phenotype, as classical genetics is not possible with uniparentally inherited organelle genes and mitochondrial transgenesis has yet to be achieved in flowering plants. In only a few cases have these links been rigorously demonstrated, namely the identification of orf138 as the causal gene for CMS in Brassica napus through analysis of recombinant cybrid mitochondrial genomes [58] and the recent identification of CMS genes in B. napus and rice via deliberate TALEN-induced deletions in mitochondrial DNA [59] . The previous identification of orf256 as the probable cause of T-CMS in wheat was based on an observed correlation between orf256 transcript processing and male fertility across only a small number of genotypes [38] , and included no near-isogenic comparisons between male-sterile and fertile lines. We show that across a larger sample of genotypes this correlation breaks down, and that neither Rf1 nor Rf3 influence orf256 processing. The fact that both RFL79 ( Rf1 ) and RFL29a ( Rf3 ) independently affect processing of the same transcript ( orf279 ), and only that transcript (as judged by genome-wide RNA-Seq), is strong evidence that orf279 is the true cause of T-CMS. The promoter and the 5′UTR region of the orf279 gene is identical to that of the atp8 gene. As observed for other chimaeric genes [15] , the presence of a promoter and 5′UTR region from a conserved mitochondrial gene probably explains how orf279 is transcribed and translated by the mitochondrial gene expression machinery. CMS has been associated with different atp8 chimaeras in sunflower, Brassica , and carrot [14] including orf138 which causes Ogura CMS and has been widely used in breeding hybrid Brassica crops [58] , [60] . Two copies of atp8 are present in T. aestivum mitochondrial genomes [61] whereas T. timopheevii has only one functional copy of the gene encoded in its genome (Supplementary Fig. 9 ). In the T. timopheevii mitochondrial genome, atp8-1 is replaced by orf279 (Supplementary Fig. 9 ). The highly hydrophobic nature of the additional sequence in the Orf279 extension of Atp8 is typical of other CMS-associated proteins [62] , [63] and may serve to disrupt the mitochondrial inner membrane or the assembly of the ATP synthase. The identification of Rf1 and Rf3 as fertility-restorer genes and orf279 as the genetic determinant of T-CMS is an important breakthrough that can be quickly translated into applications in breeding hybrid wheat. Fertility restoration in these experiments reached 96% using transgenes with strong constitutive promoters or 93% via stacking of native Rf1 and Rf3 genes. Complete fertility restoration—ideally conferred by a single gene—is required to maximise the potential gains of F 1 hybrids over conventional wheat cultivars. Ways in which that might be achieved have become clearer after this work. Higher expression of Rf1 and/or Rf3 would be expected to improve fertility, as would improving their binding to the orf279 transcript, either of which may be achievable by rational design or mutagenesis. Alternative routes to controlling male fertility in wheat are also worth exploring. As the expression of orf279 in anthers is more effectively suppressed in T. timopheevii than in Rf1 - or Rf3 -containing T. aestivum plants, T. timopheevii may carry an additional, restorer gene that is yet to be identified. For example, the Rf4 locus, located on the short arm of chromosome 6B and believed to be derived from T. timopheevii [64] has yet to be cloned and characterised. Over the last few decades, the suitability of several other sterilising cytoplasms for hybrid wheat breeding has been explored including cytoplasms from several Aegilops species [65] and Hordeum chilense [66] . The approaches we have used here to investigate the particularly complex molecular genetics of male-fertility restoration in wheat should be applicable to these other cases, too. In addition to effective fertility control systems, alterations to wheat flower architecture in parental lines to promote cross-pollination and a better understanding of the relationship between functional haplotypes and heterosis will need to be achieved for hybrid seed production to be cost-effective in wheat [11] , [13] . The recent explosion in the availability of genomic resources and technologies provides new avenues to overcome these limitations [23] . A viable path to the development of hybrid wheat cultivars would help to improve the stagnating seed yields in one of the world’s most important staple crops and will be critical in ensuring global food security. Plant material and growth conditions R197 and R0932E are Rf1 -carrying restorer lines that were developed from the same initial wheat/ T. timopheevii interspecific cross made by J. Wilson [18] . Consequently, the R197 and R0932E Rf1 genes are identical by descent. R0934F and R0946E, Australian lines originating from a private breeding programme, and the commercial variety ‘Primepi’ carry the Rf3 gene [32] . R0934F, R0946E and Primepi carry strong Rf3 restorer alleles as compared to Chinese Spring (Groupe Limagrain internal evaluation). ‘Anapurna’, a maintainer line unable to restore T-CMS, was used as a negative control in this study. In addition, a T. timopheevii line was included as it is a fertile line expected to harbour more than one Rf gene able to restore T-type CMS [18] . In addition, for the purpose of this study, a Fielder maintainer line carrying T-CMS cytoplasm (Fielder*CMS) was developed. ‘Fielder’ is a standard line used in wheat transformation protocols as it is characterised by high transformation efficiency and tissue regeneration [39] . ‘Fielder’ seeds were obtained from The National Bioresource Project (NBRP)-WHEAT (Laboratory of Plant Genetics, Graduate School of Agriculture, Kyoto University, Japan). The Fielder*CMS plants are sterile when self-pollinated. Fielder*CMS and other wheat lines generated in this project are available (MTA required) upon request from Pascual Perez, Limagrain. Plants were grown in a glasshouse under standard wheat growth conditions (16 h of light period at 20 °C and 8 h of dark period at 15 °C with constant 60% humidity) until control grains of the wild type ‘Fielder’ cultivar reached maturity stage. For pollen staining and RNA-Seq analyses, anthers at three developmental stages (A, B, C) corresponding, respectively, to early (Feekes stage 10.5), mid (Feekes stage 10.5.1/10.5.2) and late anthesis (Feekes stage 10.5.3) [67] were collected. For RNA extraction and subsequent RNA-Seq analysis, 15 anthers per sample in three biological replicates were manually collected and immediately frozen in liquid nitrogen. For pollen staining, anthers were incubated with Alexander’s stain [68] to distinguish viable and non-viable grains and inspected under a Olympus BX51 microscope (Olympus, Tokyo, Japan) equipped with a ColorView IIIu CCD camera (Olympus, Tokyo, Japan) using analySiS getIT! v5.2 software (Olympus, Tokyo, Japan). The fertility of plants was evaluated by counting the number of seeds per spike and per spikelet and comparing with the wild type Fielder and Fielder*CMS control plants. Fine mapping of the genomic regions harbouring Rf1 and Rf3 restorer genes We analysed three F 2 mapping populations (R197xKalahari, R204xAlixan and R0932ExAltigo) segregating for Rf1 and comprising 210, 218 and 212 individuals, respectively, to place the Rf1 locus between 4.0 and 10.9 cM on chromosome 1A. The largest possible interval defined by the three mapping populations is delimited by the single-nucleotide polymorphism (SNP) markers cfn1087371 and cfn0530841 (Supplementary Table 1 , Fig. 1a ). Subsequent analysis of individual F 2 recombinant plants or derived F 3 families narrowed down the Rf1 interval to between 7.0 and 8.9 cM and physically delimited the region by the SNP markers cfn1082074 and cfn0523990 (Supplementary Table 1 , Fig. 1a ). These markers were anchored to the genome sequence using the IWGSC RefSeq v1.0 reference genome [23] . Subsequently, the Rf1 locus was fine-mapped by screening 2976 and 3072 F 3 lines from R197xKalahari and R204xAlixan, respectively, derived from F 2 plants heterozygous for Rf1 . Analysis of the progenies of recombinant plants redefined the Rf1 interval to an even shorter region between 7.5 and 8.8 cM, delimited by the cfn0522096 and cfn0527067 SNP markers (Supplementary Table 1 , Fig. 1a ). To map the Rf3 locus, three F 2 mapping populations (TJB155xAnapurna, 2852xAltamira and AH46xR0946E) segregating for Rf3 and comprising 217, 135 and 246 individuals, respectively, plus a doubled-haploid (DH) population (H46xR0934F) consisting of 140 individuals were phenotyped and genotyped as described above. Rf3 was first mapped on the short arm of chromosome 1B between 18.9 and 24.2 cM on a consensus map, with the Rf3 interval physically delimited by the SNP markers cfn0554333 and cfn0560679 (Fig. 1b ). Subsequently, a joint analysis of F 3 families genetically delimited the locus between 22.2 and 22.7 cM and physically mapped the Rf3 interval between SNP markers cfn1249269 and BS00090770 (Fig. 1b ). By using the IWGSC RefSeq v1.0 assembly the left border (cfn1249269) of the Rf3 interval was anchored on IWGSCWGAV02_1BS_scaffold35219 and the right border (BS00090770) was anchored on IWGSCWGAV02_1BS_scaffold5117 (Fig. 1b , Supplementary Table 1 ). RFL capture To design bait oligonucleotides, 33 cereal genome sequences and two transcriptome data sets were screened for open reading frames (ORFs) in six-frame translations with the getorf programme of the EMBOSS 6.6.0 package [69] using parameters -minsize 279 -find 0 -reverse true. Predicted ORFs longer than 93 codons were screened for the presence of P- and PLS-class pentatricopeptide repeat (PPR) motifs using hmmsearch (with parameters -E 0.1 --domE 100) from the HMMER v3.1b1 package (hmmer.org) and hidden Markov models defined by hmmbuild [70] . HMMER output was processed using PPRfinder [71] ( https://github.com/ian-small/PPRfinder ) to identify the most likely motif arrangements in each protein. Sequences containing 10 or more P-class PPR motifs were retained for further analysis, as RFL genes are generally comprised of tandem arrays of 15–20 P-class PPR motifs [51] . For identification of RFL sequences among the P-class PPRs, the OrthoMCL algorithm [72] was used via the OrthoMCL-DB website (Release 5, 23rd July 2015) ( http://www.orthomcl.org/orthomcl/ ) to assign P-class PPR proteins from each data set into clusters. The resulting output files were screened for groups containing 49 reference RFLs [51] . In total, 633 RFL sequences were identified in the 35 cereal data sets by OrthoMCL analysis. In addition, WGS data sets of 44 sorghum accessions including landraces and wild relatives [73] were analysed in the same way and 517 additional RFL sequences identified. These 1199 RFL sequences underwent a pre-treatment process that included masking of sequences matching wheat organelle genome sequences (GenBank accessions NC_007579.1 and AB042240) as well as repeated elements of the wheat genome using the MIPS Repeat Elements Database v9.3 [74] , the TREP Repeat Elements Database v10 [75] , the TIGR Repeat Elements Database V4 [76] and RepeatMasker v.3.3.0 software ( http://www.repeatmasker.org/ ). The remaining RFL sequences were used for capture probe design with a frequency masking algorithm intended to rule out probes that match with high copy number sequences in the targeted genome(s). A set of 62,579 DNA probes ranging from 50 to 95 nucleotides were designed. On average, probes were tiled every 36 bp on the targets. The final probes were synthetized as a probe pool. Seeds of each accession were sown and plantlets were grown in etiolated conditions. After extraction using a Nucleospin Plant II kit (Macherey-Nagel, Düren, Germany) according to the manufacturer’s recommendations, DNA samples were fragmented using a Covaris (Woburn, Massachusetts, USA) device to generate a population of fragments centred around 600 bp. Sequencing libraries were prepared with KAPA Biosystems chemistry (KAPA HTP Library Preparation Kit Illumina 96 Rxn; Roche, Basel, Switzerland) according to the manufacturer’s recommendations. The libraries were then specifically enriched in RFL sequences using the probe pool (SeqCap EZ Developer Library, 12 Reactions; Roche) and two consecutive rounds of sequence capture, referred to as the double capture protocol, as recommended by the manufacturer in case of limited cumulated size of the targets in the genome. The efficiency of the capture was confirmed via the measurement of targeted sequence enrichment and untargeted sequence depletion (chloroplast genome sequence) using qPCR and primer sequences given in Supplementary Table 6 . Ultimately libraries were pooled and sequenced in paired-end mode with 300 nt read length on an Illumina MiSeq platform (Illumina, San Diego, California, USA). Overlapping paired reads were merged into a single sequence (to maximise read length) using bbmerge from the bbmap package v.35.x ( https://sourceforge.net/projects/bbmap/ ) with the parameters qtrim2 = t trimq = 10,15,20 minq = 12 mininsert = 150. Read pairs that could not be merged were discarded. The merged reads were downsampled to 300,000 reads using reformat.sh in the bbmap package (samplereadstarget = 300000). The merged and downsampled reads were assembled with the de novo assembler included in Geneious 8 (set to Medium Sensitivity/Fast) ( http://www.geneious.com/ ). Finally, contigs composed of more than 100 merged reads were retained for further analysis, with most of these composed of over 1000 reads. Sequences encoding RFL proteins were identified within these contigs as described at the beginning of this section. Finally, to identify putatively orthologous RFL sequences across all eight accessions and T. timopheevii , the 2022 RFL ORFs (Supplementary Table 4 ) were clustered using CD-HIT [36] (settings -c 0.96 -n 5 -G 0 -d 0 -AS 60 -A 105 -g 1). Cloning of candidate genes and Agrobacterium -mediated transformation RFL79 derived from R197 (sequence: R197.300k_Assembly_Contig_120_1), RFL104 sequence derived from R0932E (sequence: R0932E.300k_Assembly_Contig_82_1), RFL29a sequence derived from R0934F (sequence: R0934F.300k_Assembly_Contig_78_1), RFL29b derived from Chinese Spring (sequence: TraesCS1B02G038500.1) were cloned via a Golden Gate reaction into the destination binary plasmid pBIOS10746. The coding sequences of the candidate genes were cloned between the strong Zea mays ubiquitin promoter ( ZmUbi ) sequence containing the first intron and the SbHSP terminator (3′-UTR) from the Sorghum bicolor Sb03g006880 gene encoding a heat shock protein (HSP18.2). The screening cassette consists of the T. aestivum HMWG promoter, ZsGreen (green fluorescent protein derived from Zoanthus ) and tNos terminator sequence. The selection cassette consists of a rice actin gene promoter and first intron, the bialaphos resistance ( Bar ) gene and tNos terminator sequence. DNA fragments corresponding to the screening cassette and to the selection cassette were purchased from GenScript (Piscataway, New Jersey, USA) and used to create destination vectors. In parallel, the coding sequences of the candidates were cloned via restriction enzyme reaction, between the native T. aestivum promoter and 3′-UTRs into the destination binary plasmid pBIOS10747. The promoter sequences were obtained either from available BAC clones ( RFL29a ), from the IWGSC RefSeq v1.0 sequence ( RFL29b ) or generated by using several rounds of sequence capture protocol [77] . The corresponding sequences were synthesized by GenScript. For the RFL29a + RFL79 double construct, the coding sequences of RFL29a and RFL79 were cloned under the control of their endogenous promoters and terminators into the pBIOS10747 plasmid. The binary destination vectors pBIOS10746 and pBIOS10747 are a derivative of the binary vector pMRT [78] . All binary plasmids described above were transformed into Agrobacterium EHA105. Fielder*CMS as well as conventional Fielder cultivar were transformed with these Agrobacterium strains as described by ref. [39] . Transgenic events were generated for each of the constructs. For the ZmMac2 experiments, the ZmMac2::Barnase cassette was cloned as a Kpn I fragment from the ZmMac2::Barnase vector [40] into the Kpn I site of an pSB11-based plant binary transformation vector (pGB53) [79] . This construct was used to transform NB1 wheat [80] . The ZmMac2 sequence was synthesized with suitable restriction sites by GenScript and then cloned with the RFL29a coding sequence and the SbHSP 3′-UTR via a Golden Gate reaction into a derivative of the binary plasmid pBIOS10746. The corresponding T-DNA is described in Fig. 4a . The SbHSP 3′-UTR was replaced by that of RFL29a by restriction cloning (exchange of a Sna BI -Asc I fragment) to create the ZmMac2::RFL29a::RFL29a cassette (Fig. 4a ). These binary plasmids were then transferred into Agrobacterium EHA105 and used to transform Fielder*CMS as described above. Genotyping of Rf1 and Rf3 transformants For each plant, genomic DNA was isolated using 50 mg of fresh leaf material with a microextraction method with the DNeasy 96 Plant kit (Qiagen, Hilden, Germany) following the manufacturer’s instructions. Real-time PCR was carried out in 384-well reaction plates to estimate the number of transgenes integrated per plant. Reactions were multiplexed to simultaneously amplify the Selection Cassette Bar transgene and the endogenous gene GaMyb (GenBank accession numbers EF114937.1, EF114922.1, EF114913.1). For each sample, the reaction mixture contained 5 μL 2x TaqMan Genotyping Master mix (Applied Biosystems, Foster City, California, USA), 500 nM of each primer, 200 nM of each probe and 2 μL of genomic DNA (5–10 ng) in a final volume of 10 μL. Two replicates were performed for each sample and a calibrator sample (known 1 copy of Bar control). The PCR was run on a 7900HT Real-Time System (Applied Biosystems) using the following thermal cycling conditions: 2 min at 50 °C, 10 min at 95 °C and 40 cycles with 15 s at 95 °C and 1 min at 60 °C. Results were analysed with SDS Software v2.4 (Applied Biosystems) to estimate transgene copy number applying the 2 −ΔΔCT method [81] . Primers and probes were designed using the Primer Express software v2.0 (Applied Biosystems) and are listed in Supplementary Table 6 . An expression value of ~1 indicates single insertion of the transgene whereas a value higher than 1 indicates multiple insertions. RNA analyses RNA was extracted from plants with an RNeasy Plant Mini Kit (Qiagen) according to the manufacturer’s instructions and treated with TURBO™ DNase (Invitrogen, Carlsbad, California, USA). For orf256 and orf279 expression analyses, cDNA was synthesized using Superscript III (Invitrogen) and random primers (Invitrogen). The amplification was performed with the gene-specific primers listed in Supplementary Table 6 . Northern blotting was performed as previously described [82] . In short, 5–10 μg of total RNA per sample were separated on a 1.2% denaturing agarose gel and transferred onto Amersham Hybond N + membrane (Cytiva, formerly GE Healthcare Life Sciences, Marlborough, Massachusetts, USA). DNA fragments corresponding to a part of the coding sequence of orf256 were amplified from cDNA of T. timopheevii using primers listed in Supplementary Table 6 and cloned into pGEM‐T Easy vector (Promega, Madison, Wisconsin, USA). Positive clones served as a template for in vitro transcription using Biotin-14-CTP (Invitrogen) following the protocol supplied with the MAXIscript® In Vitro Transcription Kit (Invitrogen). Pre‐hybridization of the membrane was carried out at 65 °C for 1 h in PerfectHyb Plus Hybridization Buffer (MilliporeSigma, formerly known as Sigma-Aldrich, Burlington, Massachusetts, USA). Hybridization with RNA probes was carried out overnight at 65 °C in a fresh aliquot of the hybridisation buffer. Three 15‐min washes at 37 °C in 2× saline-sodium citrate (SSC)/0.1% sodium dodecyl sulfate (SDS), 1×SSC/0.1% SDS and 0.5×SSC/0.1% SDS, respectively, were performed. The signal of the probes was detected using the Thermo Scientific Pierce Chemiluminescent Nucleic Acid Detection Module Kit (Thermo Fisher Scientific, Waltham, Massachusetts, USA) and recorded using GE ImageQuant‐RT ECL Imager (Cytiva). One microgram of total RNA was used for cDNA synthesis and amplification of 5′ ends using the SMARTer RACE 5′/3′ Kit (Takara Bio, Kusatsu, Shiga, Japan) following the manufacturer’s instructions. PCR products were gel-eluted, cloned into pGEM‐T Easy vector (Promega) and sequenced at Macrogen (Seoul, South Korea). Gene-specific primer sequences (GSPs) are given in Supplementary Table 6 . RNA-Seq libraries were made with the TruSeq Stranded Total RNA with Ribo-Zero Plant Prep Kit (Illumina) and sequenced on a HiSeq 4000 or NovaSeq 6000 platform (Illumina) with 100 or 150 nt paired-end reads at Novogene (Novogene, China). Reads were adapter-trimmed with bbduk (parameters ktrim = r k = 23 mink = 11 hdist = 1 tpe tbo ftm = 5). Salmon (v1.3.0) [83] was used to assign reads to transcripts and calculate transcripts per million values. For nuclear/cytosolic transcripts, the IWGSC 1.1 annotations were used as a reference, but with the Chinese Spring RFL transcripts replaced by captured RFL sequences from the sequenced genotype. For mitochondrial transcripts, annotated coding sequences from the T. timopheevii mitochondrial genome (NC_022714) were used, supplemented with ten T. timopheevii -specific ORFs of over 100 codons. Where relative gene expression was evaluated (Fig. 2f ), read counts were normalised across samples using the pseudoreference approach of DeSeq2 [84] . For analysis of read coverage, adapter-trimmed reads were mapped to the T. timopheevii mitochondrial genome (NC_022714) with bbmap [85] . Multi-mapped reads were distributed randomly between the best-matching sites and rRNA regions were masked (because rRNA depletion was inconsistent across samples). Regions identical to plastid DNA were masked to avoid cross-mapped plastid reads. Read coverage was normalised by dividing by mean coverage depth excluding the masked regions. Protein extraction and immunological analysis Mitochondria were enriched from 11-day-old wheat seedlings grown on vermiculite in the dark according to a previously published protocol [86] . Wheat seedlings were cut into 0.5–1 cm pieces and ground in pre-cooled mortar and pestle in grinding medium (0.3 M sucrose, 25 mM tetrasodium pyrophosphate, 2 mM ethylenediaminetetraacetic acid (EDTA), 10 mM KH 2 PO 4 and 1% polyvinylpyrrolidone-40, 1% bovine serum albumin (BSA), 10 mM ascorbic acid, pH 7.5 with H 3 PO 4 ) with addition of acid-washed sand in a cold room. The suspension was then filtered through 4 layers of Miracloth (MilliporeSigma formerly known as Millipore). The homogenate was centrifuged for 5 min at 1000 × g at 4 °C in an Avanti J-26XP centrifuge (Beckman Coulter, Brea, California, USA). The pellet was discarded and the supernatant spun down again for 20 min at 21,000 × g at 4 °C. The resulting pellet was resuspended in residual supernatant using a small paintbrush and 500 μL of 1× wash buffer (0.3 M sucrose, 10 mM TES, 0.1% BSA, pH 7.5) and layered over a 10 mL 18%/24%/50% Percoll step gradient. Percoll gradient solutions were prepared by mixing appropriate amounts of Percoll solution (Cytiva), 2× wash buffer (0.6 M sucrose, 20 mM TES, 0.2% BSA, pH 7.5) and sterile water. The tubes were balanced and centrifuged at 40,000 × g for 45 min at 4 °C with brakes off. Intact mitochondria that formed a light yellow/whitish band towards the bottom of the tube were washed twice in 1× wash buffer and centrifuged for 20 min at 21,000 × g at 4 °C. When the available plant material was scarce, the Percoll gradient purification step was omitted and pellets after the second centrifugation step were washed in 1× wash buffer and used directly for further analyses. After the washing step, the mitochondrial pellets were resuspended in ACA buffer (0.75 M aminocaproic acid, 0.5 mM EDTA, 50 mM Bis-Tris pH 7.0) and treated with 1% n -dodecyl-β-d-maltoside solution to release membrane-bound proteins for 20 min on ice. After a 10 min-centrifugation step at 20,800 × g the supernatant was transferred into a new tube and mixed with 4 volumes of acetone supplemented with 1% β-mercaptoethanol to precipitate the proteins. After 10 min centrifugation step at 20,800 × g the proteins were resuspended directly in protein loading buffer (1 M Tris-HCl pH 6.8, 2% SDS, 10% glycerol, 0.0006% bromophenol blue, 5% β-mercaptoethanol), heated at 95 °C for 10 min and separated on a 15% Stain-Free™ SDS-PAGE gel (Bio-Rad, Hercules, California, USA). The transfer onto Amersham PVDF blotting membrane (Cytiva) was performed using a semi-dry blot apparatus (Bio-Rad). The antibody against recombinant Orf279 protein was custom-made at GenScript. Part of the unique region of Orf279 encompassing amino acid residues 137–279 was overexpressed in E. coli and used for immunisation of two rabbits. For immunological detection the anti-Orf279 antibody was diluted 1:500 and the anti‐rabbit antibodies conjugated to horseradish peroxidase (MilliporeSigma) were diluted 1:10,000 in TBST (Tris-buffered saline, 0.1% Tween 20) buffer. The chemiluminescent signals were detected with Clarity Western ECL Substrate (Bio-Rad) in an ImageQuant-RT ECL Imager (Cytiva). RNA electrophoretic mobility shift assay Recombinant RFL79 and RFL29a proteins were expressed as maltose-binding protein-fusions and purified by affinity chromatography as described previously for other PPR proteins [87] . The coding sequences of RL79 and RFL29a were amplified from genomic DNA using the PrimeStar HS DNA polymerase (Takara Bio) with primers containing attB sites for Gateway cloning technology (Invitrogen) (Supplementary Table 6 ). The obtained PCR products were subcloned into pDONR207 vector (Invitrogen) with Gateway BP Clonase II enzyme mix (Invitrogen). The positive clones were identified by sequencing at Macrogen and cloned into the expression vector pETG-41K (EMBL, Heidelberg, Germany) with Gateway LR Clonase II enzyme mix (Invitrogen). The pETG-41K vector allows an addition of 6xhistidine (His) tag that can be used for Ni-NTA purification and an MBP (maltose-binding protein) tag at the N-terminus of the recombinant protein. For protein expression, the chemically competent cells of E. coli C41(DE3) strain (MilliporeSigma) were used. Transformed cells were grown in 500 mL LB (1× Luria-Bertani and 50 mM Tris-HCl, pH 8.0) medium at 37 °C and 220 rpm until the OD 600 reached 0.4. Glass flasks with the cultures were then transferred on ice for 15 min and protein expression was initiated by addition of isopropyl β-d-1-thiogalactopyranoside (Promega) to a final concentration of 0.1 mM. The cultures were grown at 16 °C and 220 rpm overnight and harvested by centrifugation at 3000 × g for 15 min in an Avanti J-26XP centrifuge (Beckman Coulter). Bacterial pellets were dissolved in 35 mL of lysis buffer (0.5 M NaCl, 50 mM HEPES-KOH pH 8, 10 mM imidazole, and 7 mM β-mercaptoethanol) and cells were disrupted by homogenization with Avestin Emulsiflex C5 (Avestin, Ottawa, Ontario, Canada). Soluble protein fractions were cleared from cell debris by centrifugation for 15 min at 13,000 × g at 4 °C, incubated with Profinity IMAC Ni-charged resin (Bio-Rad) on a rotating wheel for 1 h and packed into empty Econo-Pac gravity columns (Bio-Rad). After three washes with 1x wash buffer (0.5 M NaCl, 50 mM HEPES-KOH pH 8, 7 mM β-mercaptoethanol, 20 mM imidazole) proteins were eluted from the Ni-charged resin with elution buffer (0.5 M NaCl, 50 mM Tris-HCl, pH 8, 250 mM imidazole) and dialysed overnight at 4 °C in dialysis buffer (0.5 M NaCl, 50 mM Tris-HCl, pH 8, 50% glycerol, 2 mM EDTA, 7 mM β-mercaptoethanol) with slow stirring on a magnetic mixer. The concentrations of the dialysed proteins were measured at ND-1000 NanoDrop spectrophotometer (Thermo Fisher Scientific). More details on protein purification and analysis are given in Supplementary Fig. 7 . The sequences of fluorescein-labelled oligonucleotides used in the REMSAs performed following the previously published protocol [87] are listed in Supplementary Table 6 . Briefly, 10 μL of binding buffer consisting of 1× THE (34 mM Tris, 66 mM HEPES, 0.1 mM EDTA pH 8), 0.2 M NaCl, 5 mM dithiothreitol, 5 mg/mL heparin, 0.1 mg/mL BSA, and 8 units of RNaseOUT (Invitrogen) were mixed with 5 μL of dialysed-protein dilution and incubated at room temperature for 10 min. The 5′-fluorescein-labelled probes (MilliporeSigma) were heated for 2 min at 94 °C and incubated on ice for at least 4 min. 10 μL of denatured probes were added to the 15 μL binding reaction for a total reaction volume of 25 μL and incubated at 25 °C for 15 min. 15 μL of the binding reaction were loaded onto a pre-run 5% native polyacrylamide gel using the 1× THE as a running buffer in a cold room. After the run gels were imaged with a Typhoon Biomolecular Imager (Cytiva). Fluorescein-labelled probes were excited by a 488 nm laser and detected through a 520 nm band-pass emission filter. Reporting summary Further information on experimental design is available in the Nature Research Reporting Summary linked to this paper.